Majorana modes andp-wave superfluids for fermionic atoms in optical lattices The quest for realization of non-Abelian phases of matter, driven by their possible use in fault-tolerant topological quantum computing, has been spearheaded by recent developments in p -wave superconductors. The chiral p x + ip y -wave superconductor in two-dimensions exhibiting Majorana modes provides the simplest phase supporting non-Abelian quasiparticles and can be seen as the blueprint of fractional topological order. Alternatively, Kitaev’s Majorana wire has emerged as an ideal toy model to understand Majorana modes. Here we present a way to make the transition from Kitaev's Majorana wires to two-dimensional p -wave superconductors in a system with cold atomic gases in an optical lattice. The main idea is based on an approach to generate p -wave interactions by coupling orbital degrees of freedom with strong s -wave interactions. We demonstrate how this design can induce Majorana modes at edge dislocations in the optical lattice, and we provide an experimentally feasible protocol for the observation of the non-Abelian statistics. Candidates for topological phases supporting non-Abelian anyons [1] with potential application in topological quantum computing [2] , [3] are found among a variety of systems including superfluid 3 He-A (ref. 4 ), the layered superconductor Sr 2 Ru O 4 (ref. 5 ), the fractional quantum Hall state at (refs 6 , 7 ) and superconductor/topological insulator or similar heterostructures [8] , [9] , [10] , [11] . Most recently, indium antimonide nano-wires in contact with an s -wave superconductor have shown promising experimental evidence consistent with the presence of the sought-after non-Abelian zero-energy Majorana states [12] , [13] . However, many questions still ask for a definitive answer. Alongside the tremendous progress in solid-state systems, cold atomic gases provide a different angle when looking at p -wave superconductors. Thanks to their largely different strengths and shortcomings compared with solid-state systems, cold atomic gases might offer solutions to problems that are yet hard to address otherwise. For instance, it is well-known that the spatial dimension of a setup can easily be controlled by optical lattices, while Feshbach resonances allow one to tune the interaction strength almost at will [14] . Unfortunately, the lifetime of p -wave resonant gases was found to be very limited [15] , [16] due to a number of well-understood decay channels [17] , [18] . Identifying realizations of atomic p -wave superfluids with a sufficient lifetime emerged as a central challenge in this field. This led to proposals such as Bose–Fermi mixtures in optical lattices [19] , [20] , [21] , microwave dressed polar molecules [22] , the introduction of synthetic spin-orbit coupling [23] , [24] , [25] , [26] , the quantum Zeno effect [27] or driven dissipation [28] . However, the complexity in these proposed setups has so far precluded an experimental realization. Here we present a simple approach to create a strong p -wave interaction for fermions in an optical lattice. The main idea is based on a resonant coupling from the lattice sites to a molecular state residing in the center of the plaquette in analogy to refs 29 , 30 . The crucial step is that the combination of a lattice setup with different orbital states and s -wave interactions can give rise to a strong induced p -wave pairing; similar ideas have recently been proposed [31] . We will demonstrate the appearance of p -wave superfluid phases via this coupling. Moreover, a setup intrinsically based on an optical lattice allows one to naturally explore the transition from a two-dimensional (2D) p -wave superfluid to Kitaev's Majorana wire [32] . Hence we identify different topological transitions [33] , where the combination of the Fermi surface topology with the symmetry of the p -wave superfluid order parameter gives rise to a rich phase diagram. Most remarkably, we find the appearance of Majorana modes localized at edge dislocations; such edge dislocations correspond to vortices in the phase of the lasers generating the lattice. In combination with another realistic ingredient to modern cold atoms experiments, single site addressability in the lattice [34] , [35] , we provide a protocol for the observation of the non-Abelian braiding statistics. Effective Hamiltonian We start with the presentation of the Hamiltonian underlying our system. We focus on a setup of spinless fermionic atoms in an optical square lattice. Then, the Hamiltonian is well-described by the tight-binding model Here and c i denote the fermionic creation (annihilation) operators at lattice site i , while μ is the chemical potential fixing the average particle number and t ij denotes the hopping energy between the nearest neighbour sites ‹ ij ›. To study the transition from a bulk 2D setup to weakly coupled one-dimensional (1D) chains, we allow for an anisotropic hopping t ij , where t ij = t x ( y ) for hopping along a link in the x-(y-)direction, respectively. The interaction between the fermions is driven by resonant couplings H x ( y ) to two distinct lattice bound states X p and Y p residing in the center of each plaquette as shown in Fig. 1 ; similar setups for bosonic atoms have been previously proposed [29] . Such a coupling is very similar to the well-known two channel model for Feshbach resonances, however, the molecular state only exists due to the presence of the optical lattice, and is localized in space. For spinless fermions on the lattice sites, these bound states must exhibit an odd parity symmetry for a non-vanishing interaction, which in our situation is a twofold degenerate p -wave symmetry. 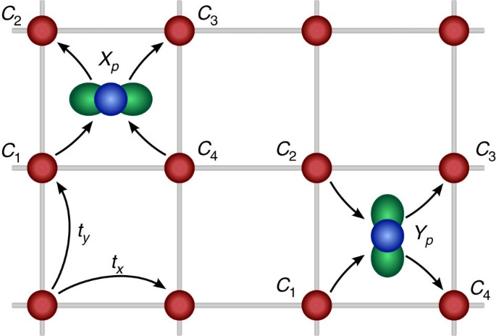Figure 1: Lattice setup. Spinless fermions residing at the lattice sites are coupled to a molecular state in the center of each plaquette. The molecular states exhibit ap-wave symmetry and are doubly degenerate. Anisotropic hoppingsty/txallow for the transition from coupled wires to the 2D isotropic system. Then, the coupling Hamiltonians reduce to Figure 1: Lattice setup. Spinless fermions residing at the lattice sites are coupled to a molecular state in the center of each plaquette. The molecular states exhibit a p -wave symmetry and are doubly degenerate. Anisotropic hoppings t y / t x allow for the transition from coupled wires to the 2D isotropic system. Full size image where the summation ∑ p runs over all plaquettes. The four lattice sites surrounding each plaquette are labelled as shown in Fig. 1 . The couplings to the lattice bound states respect the p -wave symmetry with coupling strength g , while the detuning from resonance is given by . The latter quantity also includes the chemical potential with the energy difference between the molecular state and two free fermions. The most crucial part is the possibility to induce a strong p -wave interaction by the combination of orbital degrees of freedom and s -wave interactions. Here we provide a sketch of this fundamental idea (for details we refer to the methods section): the two-particle states X p and Y p in the center of the plaquette consist of two orbital states in the optical lattice forming a repulsively bound state [36] . For these lattice molecules to fulfil the p -wave symmetry, we choose the lowest ( s -wave) and the first excited ( p -wave) state in the lattice confining the atoms in the center of the plaquette. Furthermore, the two fermions in the two orbital states have to be in different hyperfine states to profit from a stable s -wave interaction, which can be tuned by conventional Feshbach resonances [37] . This requires the coupling to the plaquette states to induce transitions between hyperfine states. To summarize: the s -wave interaction leads to the formation of repulsively bound pairs, while the orbital degree of freedom is responsible for the p -wave character of these lattice bound molecules. It is via this mechanism that the optical lattice breaks rotational symmetry and couples to states with different orbital symmetry allowing for the conversion of s -wave to p -wave interactions. Mean-field theory We first study the zero temperature phase diagram within mean-field theory. Such a mean-field analysis is well-justified as recent density matrix renormalization group simulations [30] have demonstrated the appearance of a p -wave superfluid exhibiting Majorana modes in a double wire setup. The authors of ref. 30 studied a similar interaction between the wires, and demonstrated the qualitative agreement with the mean-field theory predictions. Using density matrix renormalization group simulations, we verified that this qualitative behaviour remains valid also for three-wires for our effective Hamiltonian. As we are here interested in a higher dimensional setup, we expect that the influence of thermal and quantum fluctuations are even further suppressed and the phase diagram is again well-captured within mean-field theory. The resonant coupling between the fermions and the molecular state gives rise to a p -wave pairing for the fermions and leads to a p -wave superfluid. Within mean-field theory the superfluid order parameters take the form Δ x =4 g ‹∑ p X p ›/ N and Δ y =4 g ‹∑ p Y p ›/ N , and describe the macroscopic occupation of the zero momentum mode for the molecular states. Then, the Hamiltonian reduces to a quadratic fermionic theory Here , and N denotes the number of lattice sites. accounts for the conventional operator-independent parts. Furthermore, the tight-binding dispersion for the fermions reduces to , while the gap parameter takes the form of a p -wave superfluid where a denotes the lattice spacing. Using a Bogoliubov transformation, we obtain the superfluid excitation spectrum , and the ground-state energy per unit cell with denoting the volume of the first Brillouin zone. The order parameters Δ x and Δ y are determined by the gap equation minimizing the ground-state energy The results of the mean-field theory are shown in Fig. 2b : we find a p x + ip y superfluid for the fully isotropic setup with t x = t y where Δ x =± i Δ y . In addition to the U (1) symmetry breaking, this phase also breaks time-reversal symmetry. For finite interaction strength the p x + ip y superfluid is stable to a small anisotropy in the hopping. Note that the anisotropic behaviour is reflected in the order parameter, that is, |Δ x |≠|Δ y |. However, we denote a p x + ip y superfluid as a phase with a finite order parameter Δ x and Δ y obeying the fixed phase relation Δ x /Δ y =± i |Δ x /Δ y |. For increasing anisotropy t x ≠ t y , transitions into a p x ( p y ) superfluid can appear, depending on the value of the chemical potential μ . 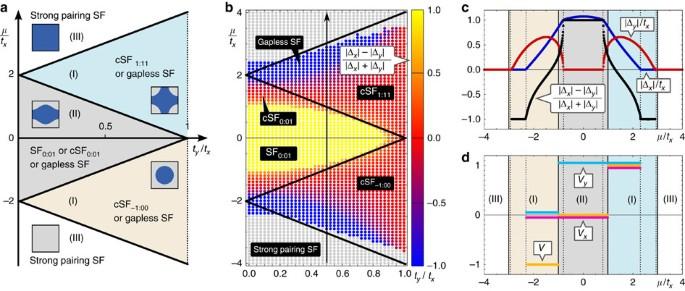Figure 2: Topological phases and mean-field phase diagram. (a) Topological phase diagram: we can distinguish between three different topological regions. However, the topological indices also depend on the order parameter of the superfluid (see main text). The different phases are denoted asfor time-reversal invariant andfor chiral superfluids withνthe strong topological index andthe weak ones. The pictorial insets show the topology of the Fermi surface within each phase. (b) Mean-field phase diagram for: for the rotationally symmetric setup withtx=tythe ground state is given by apx+ipysuperfluid, while for strong anisotropytx≠tya purepxorpysuperfluid order parameter dominates. The grey dots mark the points where the gap parameters are too small for a convergence of the numerical calculations, and therefore no superfluid phase is accessible for experimentally realistic temperatures. (c,d) Show the gap parameters |Δx|/tx, |Δy|/txand (|Δx|−|Δy|)/(|Δx|+|Δy|) along a cut through the phase diagram atty=tx/2 (see arrow inb), as well as the different topological indices. The colour shading corresponds to the topological classification ina, solid (dashed) lines indicate the topological (mean-field) transitions. It is important to stress, that the topological indexνyjumps to 1 at a different position than the vanishing of Δy(cf.candd), that is, the topological transitions are essentially decoupled from the mean-field transitions. Figure 2: Topological phases and mean-field phase diagram. ( a ) Topological phase diagram: we can distinguish between three different topological regions. However, the topological indices also depend on the order parameter of the superfluid (see main text). The different phases are denoted as for time-reversal invariant and for chiral superfluids with ν the strong topological index and the weak ones. The pictorial insets show the topology of the Fermi surface within each phase. ( b ) Mean-field phase diagram for : for the rotationally symmetric setup with t x = t y the ground state is given by a p x + ip y superfluid, while for strong anisotropy t x ≠ t y a pure p x or p y superfluid order parameter dominates. The grey dots mark the points where the gap parameters are too small for a convergence of the numerical calculations, and therefore no superfluid phase is accessible for experimentally realistic temperatures. ( c , d ) Show the gap parameters |Δ x |/ t x , |Δ y |/ t x and (|Δ x |−|Δ y |)/(|Δ x |+|Δ y |) along a cut through the phase diagram at t y = t x /2 (see arrow in b ), as well as the different topological indices. The colour shading corresponds to the topological classification in a , solid (dashed) lines indicate the topological (mean-field) transitions. It is important to stress, that the topological index ν y jumps to 1 at a different position than the vanishing of Δ y ( cf . c and d ), that is, the topological transitions are essentially decoupled from the mean-field transitions. Full size image Finally, we point out that at zero temperature true long-range order as predicted within mean-field theory survives, while thermal fluctuations will lead to (quasi) long-range order for our 2D setup. Here we are mainly interested in the topological properties of the system, which are not affected by these phase fluctuations of the order parameter. Topological phase transitions In addition to the mean-field transitions, the lattice system also exhibits a series of topological quantum phase transitions beyond those found in the classification of continuum 2D superfluids [38] . These topological properties are most conveniently studied by analyzing the quadratic Hamiltonian in equation (3), where the superfluid order parameters Δ x and Δ y determine the symmetries. In the parameter regime, where the superfluid exhibits an excitation gap, the topological properties are characterized by three topological indices [33] ; see the methods section for a simple method to determine the topological indices in our setup. The first one denotes the strong topological index given by the Chern number ν characterizing the 2D p x + ip y superfluid, and takes values , see Fig. 2a . In addition, the system exhibits two weak topological indices [39] , [40] , which we denote as and . The latter quantities are the topological indices, which characterize the appearance of Majorana modes in Kitaev's Majorana wire [32] , and can be finite in p x superfluids as well as chiral p x + ip y superfluids. It is important to stress that the phase boundaries for the topological phase transitions are independent of the strength of the superfluid order parameters, and they only depend on the topology of the Fermi surface. Therefore, we can distinguish between three different regions, see Fig. 2a : region (I) with a closed Fermi surface, region (II) with an open Fermi surface and finally the strong pairing regime (III), where in absence of interactions the system is in a trivial band insulating (vacuum) state. In the latter region (III), the superfluids exhibit no topological order with ; thus it is not of interest in the following. The combination of the topological indices with the superfluid order parameter allows us now to characterize the different phases. We use the notation for time-reversal invariant superfluids and for chiral superfluids. First, we start with the chiral p x + ip x superfluid. Here we obtain two fundamentally different topological phases, see Fig. 2a : (I) the strong topological superfluids cSF −1:00 and cSF 1:11 with a finite Chern number . Within the standard symmetry classification scheme [41] , [42] , [43] , the phase is in the symmetry class D (particle–hole symmetry). It is a special property of this phase that the weak indices depend on the chemical potential, that is, we obtain for μ >0 and for μ <0. This property will strongly influence the Majorana modes, see below. In region (II), we find a weak topological superfluid in the symmetry class D (cSF 0:01 ). On the other hand, for the p x superfluid, we obtain a weak topological superfluid (SF 0:01 ) in region (II) which belongs to the class BDI, see Fig. 2a . While in the region with closed Fermi surface (I), the superfluid phase becomes gapless (that is, nodal) without any topological properties. For completeness, we point out that the p y superfluid is gapless in region (I) and (II). The full phase diagram is then obtained by combining the mean-field phase diagram in Fig. 2b with the topological properties in Fig. 2a . Its details strongly depend on the strength of the coupling parameters. Here we are mainly interested in strong couplings with with large superfluid gaps. Most remarkably, we find that for all of the above discussed topological phases are realized for varying values of μ / t x and t y / t x , see Fig. 2 . Majorana modes at edge dislocations Associated with the topological index, we expect the appearance of Majorana modes at topological defects in the system. Here such topological defects can either be vortices or—as a distinct feature of the lattice setup—also lattice dislocations. The Majorana modes are most conveniently derived as zero-energy modes of the quadratic Hamiltonian where the symmetry properties of the gap Δ ij are determined by mean-field theory. Then the spatial dependence of the gap allows to imprint vortices, while dislocations are directly implemented into the lattice structure. Generally, we expect the Majorana modes in the vortex core for Chern number , while the weak index gives rise to Majorana modes localized at lattice dislocations with Burgers vector ± e x , y . The latter can be easily understood in the limit t y =0, where the system reduces to coupled 1D wires: then, a pair of dislocations corresponds to the inclusion/removal of a 1D wire of finite length into the bulk 2D system, see Fig. 3a . This bulk superfluid induces a p -wave pairing order parameter onto this single chain realizing the ideal toy model of a single Majorana chain [32] ; this behaviour is in analogy to the proposals for the realization of Majorana modes in solid-state systems [8] , [9] . 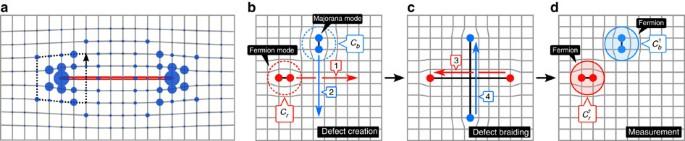Figure 3: Braiding of dislocation based Majorana modes as touchstone of non-Abelian statistics. (a) Majorana modes at lattice dislocations: an edge dislocation pair with Burgers vector ±ey(black arrow) forming a single quantum wire (red line) immersed into the bulk superfluid. For a finite weak topological indexsuch a setup generates two Majorana modes at the ends of the wire. The localized wave function of the two Majorana modes is determined by solving the quadratic theory (see equation (7)) in a parameter regime with(seeFig. 2b) on the shown lattice geometry by means of a Bogoliubov transformation. The radii of the blue circles are proportional to the square of the Majorana modes’ wave function. (b) Four Majorana modes are generated by the formation of two dislocation pairs, and then spatially separated: first along path 1 and subsequently along path 2. (c) The braiding operation is achieved by recombining the Majorana modes along path 3 and then path 4. (d) The braiding transforms the initially unoccupied state at each dislocation pair into an occupied fermion mode. The subsequent measurement of the unpaired fermions is a unique signature of the non-Abelian braiding statistics of the Majorana modes. Figure 3: Braiding of dislocation based Majorana modes as touchstone of non-Abelian statistics. ( a ) Majorana modes at lattice dislocations: an edge dislocation pair with Burgers vector ± e y (black arrow) forming a single quantum wire (red line) immersed into the bulk superfluid. For a finite weak topological index such a setup generates two Majorana modes at the ends of the wire. The localized wave function of the two Majorana modes is determined by solving the quadratic theory (see equation (7)) in a parameter regime with (see Fig. 2b ) on the shown lattice geometry by means of a Bogoliubov transformation. The radii of the blue circles are proportional to the square of the Majorana modes’ wave function. ( b ) Four Majorana modes are generated by the formation of two dislocation pairs, and then spatially separated: first along path 1 and subsequently along path 2. ( c ) The braiding operation is achieved by recombining the Majorana modes along path 3 and then path 4. ( d ) The braiding transforms the initially unoccupied state at each dislocation pair into an occupied fermion mode. The subsequent measurement of the unpaired fermions is a unique signature of the non-Abelian braiding statistics of the Majorana modes. Full size image For the verification of the presence of Majorana modes, we diagonalize the Hamiltonian (7), which can be efficiently achieved numerically; an example is illustrated in Fig. 3a . In summary, we find for the phase Majorana modes in the core of vortices. Most remarkably, the system also exhibits Majorana modes at edge dislocations e x , y , but only for positive chemical potential μ >0 with a finite weak topological index ν x = ν y =1. Similarly, the cSF 0:01 and SF 0:01 only exhibit Majorana modes at edge dislocations with Burgers vector ± e y . Nevertheless, the two phases show distinct features due to their different symmetry classification: for the chiral phase cSF 0:01 in symmetry class D, the topological index is a index. Therefore, a pair of double dislocations with Burgers vector ±2 e x , y leads to a hybridization of the Majorana modes, and consequently no ground-state degeneracy. In turn, the time-reversal symmetric phase SF 0:01 is in the symmetry class BDI, which gives rise to a topological index. Consequently, a pair of double dislocations essentially describes a two wire setup and provides four Majorana modes with a fourfold ground-state degeneracy. This behaviour is well-confirmed within the numerical solution of the Bogoliubov-de Gennes equations. The described lattice setup allows us to provide a protocol for the observation of the non-Abelian braiding statistics of the Majorana modes residing at edge dislocations. In cold atomic gases, an edge dislocation corresponds to a vortex in the optical field generating the optical lattice [44] . Such edge dislocations are most conveniently generated in a setup with local site addressability [34] , [35] , [45] , where arbitrary shapes of the lattice can be achieved. In combination with a time-dependent modulation of the masks generating the lattice, a full spatial and temporal control on edge dislocations is foreseeable in the near future. Such a setup then offers the opportunity for the observation of the non-Abelian statistics of Majorana modes by braiding the dislocations. While the braiding of vortices in a superfluid has previously been predicted for the observation of the non-Abelian statistics [46] , [47] , such experiments suffer from the difficulty to control a collective degree of freedom such as the superfluid phase, and the problem to insert adiabatically vortices into a superfluid. Here edge dislocations in the lattice are much more favourable due to the precise and simple control on the lattice structures available in cold atomic gases. In addition, the lattice eliminates the localized subgap states which occur at energies of small fractions of the bulk gap in the vortices of continuum p -wave superfluids, and which may render braiding experiments difficult to realize in neutral superfluids [48] , [49] . In the following, we present the protocol for measuring the non-Abelian statistics of the Majorana fermions, see Fig. 3b–d . It is important that all operations are performed adiabatically, that is, slower than the characteristic time scale given by the superfluid gap. In a first step, we initialize the system by adiabatically creating two dislocation pairs. At each pair, we obtain a single fermionic mode described by the operators c r , b † with a finite energy gap. This fermion mode is unoccupied as at low temperatures all fermions are Cooper paired. The next step separates the two dislocation pairs first along path 1 and then along path 2. This operation splits the fermionic modes into Majorana modes localized at the edge dislocations, and gives rise to a fourfold degenerate ground state of which two are accessible at fixed fermion number parity. However, adiabaticity of the process ensures a well-defined initial state with c r , b | g ›=0. Next, we perform the braiding by recombining the two dislocation pairs along path 3 and finally path 4. This process corresponds to moving the two Majorana modes around each other. According to the general non-Abelian braiding rules for Majorana modes [50] , this transforms the fermionic operators via ; here we drop a phase factor, which is irrelevant for the protocol. As a consequence, the initially unoccupied state becomes occupied by one fermion each, that is, . In a physical picture, the braiding operation takes one Cooper pair from the superfluid condensate and splits it into two fermions with one residing at each dislocation pair. It is the strength of the non-Abelian braiding statistics, that this characteristic signature is independent of the braiding path, as well as any dynamical phase picked up during the adiabatic motion. We tested numerically that the gap remains always on the order of the superfluid gap for the full braiding protocol. To probe the system, one ramps the energy difference of the molecular state to the free fermionic states ℏ ω to negative values, which drives the system into the strong pairing phase with all paired fermions residing in the center of the plaquettes. This procedure is the analogue to the process of forming pairs via a Feshbach resonance [36] . Finally, a measurement of the fermionic density on the original lattice sites [34] probes the unpaired fermions in the system. Here we expect one unpaired fermion at each dislocation pair. To test the protocol against induced noise, finite temperature or violation of adiabaticity, one can test the process against a background measurement with a reversed order of path 3 and 4. Since this process does not braid the two Majorana modes, no unpaired fermions should be present in an ideal experiment. In summary, we have proposed an experimentally realistic setup for the realization of a p -wave superfluid supporting Majorana fermions at lattice dislocations in a 2D optical lattice. Furthermore, we have explained how this setup allows for an efficient braiding of the Majorana fermions and might thus pave the way towards the experimental demonstration of the anyonic nature of Majorana fermions. Topological indices The topological classification of quadratic fermionic theories is based on their membership in one of the 10 Altland–Zirnbauer symmetry classes [41] , [42] , [43] . Perturbations that neither violate these symmetries nor close the gap cannot alter the topological class of the theory. In particular, there is no necessity for translational symmetry, which, in fact, is one of the peculiarities of topological phases. Nevertheless, the only viable labelling scheme for such phases makes use of topological invariants that are defined as functionals of the momentum space representation of the theory under consideration. Hence the mathematical machinery enforces us to fall back to translationally invariant theories to obtain the topological invariants (‘labels’), which then characterize the topological phases even in the case of weak disorder. The momentum space representation of our theory reads and, for a finite excitation gap E q ≠0, the Hamiltonian can be parametrized by a (normalized) Bloch vector , where denotes the vector of Pauli matrices. The Bloch vector defines a continuous mapping n : T 2 → S 2 with from the first Brillouin zone T 2 (the torus) to the Bloch sphere S 2 . The strong topological index is the integral of the Berry curvature over the Brillouin zone T 2 and given by the first Chern number It can be interpreted as the winding or Skyrmion number of the vector field as q wraps around the torus. The weak topological indices are given by the Berry phase along paths through the high symmetry points ( q x , q y )=( π ,0), ( π , π ) for ν x and (0, π ), ( π , π ) for ν y , respectively. They can be interpreted as winding numbers of about the origin, since the Bloch vector is constrained to a great circle on the paths through the high symmetry points. This winding number is easily calculated via and analogously for ν y . The strong and weak topological phases of our 2D theory are then completely classified by the triple ν : ν x ν y (ref. 33 ) which gives rise to our notation in Fig. 2 . Microscopic setup The fermionic states described by the operators reside on the sites of the optical lattice and are in the lowest Bloch band. The design of the interaction requires the coupling of these states to different internal states trapped by an optical lattice with the minima in the center of the plaquettes. Such a setup is most conveniently achieved for cold atomic gases with a metastable 3 P 2 state such as 87 Sr or 171 Yb. Then, the metastable 3 P 2 states are trapped at the sites of the lattice, while the ground state 1 S 0 is trapped in the center of the plaquette for an optical lattice close to the anti-magic wavelength. Therefore, the setup requires only a single 2D optical lattice. The experiment maintains the population of fermionic atoms on the lattice sites | i › in a single hyperfine state. Consequently, light assisted two-particle losses from the metastable 3 P 2 are quenched due to their fermionic statistic. Next, we focus on the state trapped in the center of the plaquette. We are interested in two different hyperfine states in the electronic ground state 1 S 0 , which will be denoted by a spin index σ with σ ε{↓, ↑}, and a setup with suppressed tunnelling between different plaquettes. The lowest lying state at each plaquette p exhibits s -wave symmetry and will be denoted as |0, σ › p , while the first excited state | α , σ › p with α ε{ x , y } is twofold degenerate and exhibits a p -wave symmetry, see Fig. 4b . 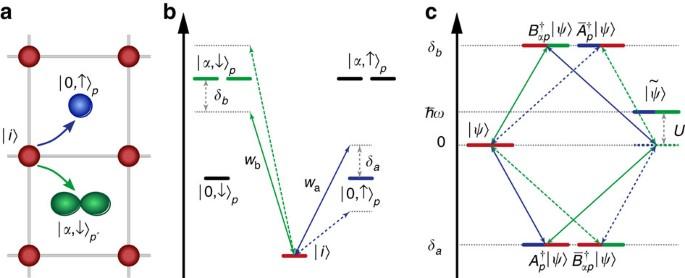Figure 4: Microscopic setup. (a) The lattice sites |i› are coupled to two different internal states trapped in the center of the plaquette. The first one |0, ↑›pexhibits ans-wave orbital symmetry, while the second one |α, ↓›pshows ap-wave symmetry and is twofold degenerate. (b) Single particle level structure with the relevant transitions (solid lines). The additional transitions (dashed lines) are required for the design of the desired coupling Hamiltonian. (c) Energy levels for the two-particle states with the two interfering paths:describes the state with two fermions on the lattice sites surrounding the plaquette, whiledescribes the near resonant repulsively bound molecule withp-wave symmetry. Figure 4: Microscopic setup. ( a ) The lattice sites | i › are coupled to two different internal states trapped in the center of the plaquette. The first one |0, ↑› p exhibits an s -wave orbital symmetry, while the second one | α , ↓› p shows a p -wave symmetry and is twofold degenerate. ( b ) Single particle level structure with the relevant transitions (solid lines). The additional transitions (dashed lines) are required for the design of the desired coupling Hamiltonian. ( c ) Energy levels for the two-particle states with the two interfering paths: describes the state with two fermions on the lattice sites surrounding the plaquette, while describes the near resonant repulsively bound molecule with p -wave symmetry. Full size image The coupling between the states on the lattice to the center of the plaquette is driven by two Raman transitions or alternatively by direct transitions. The first Raman transition with detuning δ a couples to the state |0, ↑› p providing the Hamiltonian with , and the operator creating a fermion in the state |0, ↑› p . The coupling strength w a accounts for the Rabi frequency as well as the wave function overlap. Note that the form of the coupling is determined by the s -wave symmetry of the state |0, ↑› p . In analogy, the second Raman transition couples to the states | α , ↓› p with fermionic operators and the detuning δ b . To simplify the discussion, we set δ b =− δ a and w a = w b . Then, the coupling Hamiltonian reduces to with . Note, the different couplings due to the orbital p -wave symmetry of the states | α , ↓› p . The main idea for the design of the interaction is now the fact that the state with two fermions in the center of the plaquette exhibits a strong onsite interaction U due to the s -wave scattering between two different hyperfine states. Within the rotating frame its energy is given by ℏ ω = δ a + δ b + U = U , see Fig. 4c . This motivates the introduction of two bosonic molecular states and exhibiting orbital p -wave symmetry. For a choice of the detunings with , we can then adiabatically eliminate all states with a single fermion in the center of the plaquette and arrive at the effective coupling Hamiltonian with . Note that we have omitted additional terms describing an induced hopping of the fermionic operator c i ; these terms will be discussed below. The resonant coupling of the fermionic states c i to the p -wave molecules X p and Y p residing in the center of the plaquette reduces to This coupling term differs from the desired interaction in equation (2); the last two terms describe a second representation of the p -wave symmetry for the coupling. While this coupling Hamiltonian gives rise to interesting p -wave superfluids, it is desirable to suppress these additional coupling terms. In the following, we present a scheme, which completely quenches these terms, while for an experimental realization it is sufficient to weakly suppress them. The scheme is achieved by an additional transition with opposite detunings but equal coupling strengths, where the phase is spatially varying. The main requirement on the phase is that the coupling to the state c 1 exhibits the opposite sign than the coupling to c 2 , while c 1 and c 3 have the same sign. The desired behaviour is achieved employing the principles of ref. 51 , by adding Raman lasers with a contribution of the wave vector within the plane of the optical lattice, that is, with k 0 the wave vector of the square lattice potential. By contrast, the Raman lasers for transitions must be incident at a right angle to the system. Then, we obtain the additional coupling terms and . The full coupling Hamiltonian exhibits interference between the two independent excitation channels for the molecules, see Fig. 4c , and reduces to which reveals the desired coupling in equation (2) with ℏ ω = U and . In addition, the induced hopping terms via the single excitation in the center of the plaquette reduces to an additional conventional hopping as in equation (1) with t x = t y =2| w a | 2 /δ a . Its interference with the direct hopping allows us to tune the ratios g / U and t / U independently. How to cite this article: Bühler, A. et al. Majorana modes and p -wave superfluids for fermionic atoms in optical lattices. Nat. Commun. 5:4504 doi: 10.1038/ncomms5504 (2014).